NO at low concentration can enhance the formation of highly oxygenated biogenic molecules in the atmosphere The interaction between nitrogen monoxide (NO) and organic peroxy radicals (RO 2 ) greatly impacts the formation of highly oxygenated organic molecules (HOM), the key precursors of secondary organic aerosols. It has been thought that HOM production can be significantly suppressed by NO even at low concentrations. Here, we perform dedicated experiments focusing on HOM formation from monoterpenes at low NO concentrations (0 – 82 pptv). We demonstrate that such low NO can enhance HOM production by modulating the RO 2 loss and favoring the formation of alkoxy radicals that can continue to autoxidize through isomerization. These insights suggest that HOM yields from typical boreal forest emissions can vary between 2.5%-6.5%, and HOM formation will not be completely inhibited even at high NO concentrations. Our findings challenge the notion that NO monotonically reduces HOM yields by extending the knowledge of RO 2 -NO interactions to the low-NO regime. This represents a major advance towards an accurate assessment of HOM budgets, especially in low-NO environments, which prevails in the pre-industrial atmosphere, pristine areas, and the upper boundary layer. Atmospheric aerosols are crucial to Earth’s radiative forcing and climate, yet their influence remains poorly quantified [1] . Globally, organic aerosols contribute significantly to the total aerosol mass [2] , [3] , [4] , [5] . Oxidation pathways of various volatile organic compounds (VOCs) involves autoxidation of peroxy (RO 2 ) radicals [6] . The products, known as highly oxygenated organic molecules (HOM) [7] , have recently been observed in various environments in the atmosphere. Owing to their high oxidation state and low volatility, HOM are a major source of secondary organic aerosol (SOA) [8] and contribute significantly to new particle formation (NPF) [9] , [10] , [11] . NO x concentrations are substantially elevated in the present-day atmosphere due to anthropogenic emissions. NO x profoundly influences HOM formation. First, it can regulate the atmospheric oxidation capacity and consequently affect the oxidation of VOCs [12] , [13] , [14] , [15] ; Second, NO x can greatly influence the extent of RO 2 radical autoxidation [16] and thus HOM composition by directly reacting with RO 2 radicals, leading to enhanced formation of organic nitrates and suppressed formation of HOM dimers [6] , [17] , [18] , [19] , [20] , [21] , [22] , [23] , [24] , [25] . Up to now, the second effect remains poorly quantified, presenting an important obstacle towards a complete understanding of HOM budget and its impacts on aerosol formation in the atmosphere. Currently, most laboratory experiments have been conducted either at effectively zero NO x (with very high VOC: NO x ), or at relatively high NO x concentrations. It is widely accepted that high NO x suppresses RO 2 autoxidation and HOM formation [16] . Yet, little is known about HOM formation at low but non-zero NO x concentrations (i.e., NO ranges from 5–100 pptv and NO 2 ranges from 0.1–5 ppbv), characteristic of the pre-industrial atmosphere, the pristine environments, the upper boundary layer, and likely the future atmosphere if NO x concentration continuously declines. Because the interactions between RO 2 and NO x are so complex (involving the different roles of NO, NO 2 , and NO 3 ), the overall influence on HOM formation can be highly nonlinear. Therefore, simply extrapolating the results derived from high-concentration experiments to low-concentration conditions, or even interpolating between high-NO x and effectively zero NO x , may lead to substantial biases [26] , [27] . In this work, we perform dedicated experiments at the CERN CLOUD (Cosmics Leaving Outdoor Droplets) chamber with molecular-level observations and simulations focusing on the HOM formation at low NO concentrations [28] . We demonstrate that the role of NO x in HOM formation is more nuanced than simple suppression, and low NO concentrations can cause a previously overlooked increase in HOM yields. An overview of experimental observations In the experiments, we kept the chamber conditions stable at a temperature of 278 K and 38% relative humidity. A 2:1 mixture of α-pinene and Δ−3-carene comprised the VOC precursors, representative of the typical monoterpene profile above the canopy in a boreal forest in southern Finland (the SMEAR II station, the reference site for this study) [29] , [30] . In different experiments, the steady-state mixing ratio of total monoterpenes was approximately 300, 600, and 1200 pptv. We controlled NO x in three distinct sequences: experiments with only NO 2 to represent the nighttime condition (Fig. 1a ); experiments with variable NO x concentrations with a constant NO to NO 2 ratio (~0.007) to represent the morning (Fig. 1b , c ); and experiments at constant NO x with variable NO to NO 2 ratios to represent the evolution from night to noon (Fig. 1d ). These experiments are referred to as “pure NO 2 ”, “constant NO/NO 2 ”, and “variable NO/NO 2 ” hereafter in this work. The highest NO 2 and NO mixing ratios in these experiments were 4.6 ppbv and 82 pptv, respectively. A vital feature of these experiments is the precise control and monitoring of NO and monoterpenes at low concentrations, which to the best of our knowledge, has never been achieved in previous studies. This allows us to successfully reproduce the chemical environment of the boreal forest atmosphere, and to investigate the HOM production in detail in the low-NO regime. A list of experiments illustrated in Fig. 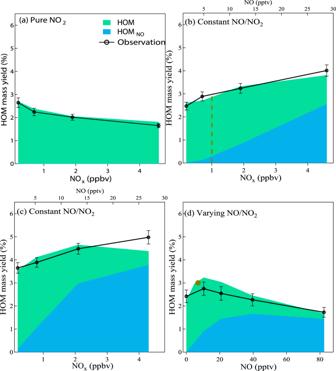Fig. 1: Comparison of measured and modelled mass yields of highly oxygenated organic molecules (HOM). In (a) a pure NO2experiment run with 1200 pptv monoterpene, (b) a constant NO/NO2experiment with 1200 pptv monoterpene, (c) a constant NO/NO2experiment with 300 pptv monoterpene and (d) a varying NO/NO2experiment with around 1 ppbv NO2and 1200 pptv monoterpene. The brown solid circle in (d) denotes the HOM mass yield obtained from the constant NO/NO2experiment with around 1 ppbv NO2and 7 pptv NO (the brown dash line in (b)). Model simulated HOM represents molecules formed without NO participation and are denoted in green; HOMNOrepresents molecules formed with NO’s involvement and are denoted in blue. The propagated error of the HOM yield varies within 6–8% among different experiments with the calculation method provided in the Methods. 1 is provided in Supplementary Table 1 , and detailed information on the experimental design and instrumentation is provided in Methods. Fig. 1: Comparison of measured and modelled mass yields of highly oxygenated organic molecules (HOM). In ( a ) a pure NO 2 experiment run with 1200 pptv monoterpene, ( b ) a constant NO/NO 2 experiment with 1200 pptv monoterpene, ( c ) a constant NO/NO 2 experiment with 300 pptv monoterpene and ( d ) a varying NO/NO 2 experiment with around 1 ppbv NO 2 and 1200 pptv monoterpene. The brown solid circle in ( d ) denotes the HOM mass yield obtained from the constant NO/NO 2 experiment with around 1 ppbv NO 2 and 7 pptv NO (the brown dash line in ( b )). Model simulated HOM represents molecules formed without NO participation and are denoted in green; HOM NO represents molecules formed with NO’s involvement and are denoted in blue. The propagated error of the HOM yield varies within 6–8% among different experiments with the calculation method provided in the Methods. Full size image A nitrate-based chemical ionization mass spectrometer (CI-APi-TOF) [6] , [31] was deployed to measure gas-phase HOM; these were classified as molecules without (CHO) and with nitrogen atoms (CHON), the latter likely being organic nitrates. We show the variations of some fingerprint CHON- and CHO- HOM for different monoterpene and NO x values in Supplementary Fig. 1 . The corresponding dependence of HOM concentrations and mass yields on NO x is illustrated in Fig. 1 and Supplementary Fig. 2a – d . The response of HOM production to NO x levels shows marked differences for different NO x sequences, indicating that NO x influences HOM formation in a complicated manner. For example, in the pure NO 2 sequence, the total HOM yield decreases monotonically as the NO 2 concentration rises (Fig. 1a ). However, in a nearly identical sequence with constant NO/NO 2 , differing only by a small amount of NO (maximum 28 pptv), HOM yields increase monotonically, from about 2.5% to 4.0% as the NO x concentration rises (Fig. 1b ). This enhancement is more pronounced at low monoterpene concentrations (Fig. 1c ) than at high monoterpene concentrations when the NO x concentration is identical. These results clearly show that the roles of NO and NO 2 in HOM formation are different – while NO 2 suppresses HOM formation monotonically [32] , NO at low concentrations can enhance HOM formation. The influence of NO on HOM yields is seen more clearly in the varying NO/NO 2 sequence; When NO increases from 0 to 82 pptv at an approximately constant NO 2 concentration near 1 ppbv, it first enhances HOM production, but as it further increases the enhancement gradually diminishes and turns into suppression (Fig. 1d ). Altogether, these observations clearly show that NO has a non-linear effect on HOM yields, challenging the notion that NO monotonically suppresses HOM production by inhibiting the autoxidation of RO 2 [15] , [16] . A mechanistic understanding of the roles of NO x in HOM formation We use the Aerosol Dynamics gas- and particle-phase chemistry model for laboratory CHAMber studies (ADCHAM) to further obtain a mechanistic understanding of the influence of NO on HOM formation [11] . This model simulates HOM formation on a molecular level. We extend the peroxy radical autoxidation mechanism (PRAM) module [11] , [33] in ADCHAM by incorporating NO 3 chemistry and refining the representation of alkoxy radical (RO) isomerization, which better describes HOM formation through the interactions between monoterpenes and NO x . As shown in Fig. 1 and Supplementary Fig. 2 , the model not only reproduces the HOM distribution at various experimental conditions, but also captures the variation of HOM concentrations for the different NO x sequences we employed in our experiments, showing that the model setup is reasonable and results are robust. With the help of ADCHAM, we track each reaction channel and divide HOM into HOM NO and HOM non-NO . HOM NO denotes HOM formation directly involving NO in at least one reaction, forming either an organic nitrate or an RO radical. HOM non-NO denotes HOM formation without any reactions involving NO. We can see that the HOM NO increase significantly in three NO-involved sequences (Fig. 1b-d ). The fraction of HOM NO is approximately 85 % at low monoterpene concentrations (Fig. 1c ) or high NO (Fig. 1d ). This high fraction of HOM NO in the model also is consistent with our PMF analysis (see Methods and Supplementary Fig. 3 ). This also agrees with our previous PMF analysis of ambient data at our reference site, where the dominant daytime factors are NO-involved (accounting for ~90% of the total HOM concentration) with around 80 pptv NO (Supplementary Fig. 4 ) [17] , suggesting NO is involved in the formation of the majority of HOM at quite low concentrations. Next, we use the varying NO/NO 2 sequence to investigate the non-linear effects of NO on HOM yields. We find two main causes. First, NO suppresses RO 2 production and slows the second-order RO 2 cross-reactions dramatically. When these cross-reactions are the dominant RO 2 sink, they can terminate RO 2 chemistry before isomerization reactions initiate autoxidation. Second, NO enhances RO formation, which also undergoes autoxidation and leads to second-generation RO 2 . Both these effects enhance HOM formation when RO 2 + NO is not the major RO 2 sink but suppress HOM formation when RO 2 + NO becomes the dominant RO 2 sink. This drives the nonlinear HOM production with a peak at low but non-zero NO. An important detail is that only some RO 2 can undergo rapid autoxidation. According to the latest understanding of bicyclic monoterpene oxidation, only a fraction of first-generation RO 2 can undergo cyclobutyl ring breaking, a necessary step for further autoxidation and formation of HOM-RO 2 [34] . This suggests a fixed yield of RO 2 that can undergo autoxidation. The non-linear effect of NO on HOM yield is essentially caused by influencing the further oxidation of these potential HOM-RO 2 (p-HOM-RO 2 , defined as RO 2 that can undergo autoxidation with n O < 7) to HOM-RO 2 (defined as RO 2 that is autoxidized to n O ≥ 7, Fig. 2b ), e.g., from C 10 H 15 O 4 to C 10 H 15 O ≥7 in the ozonolysis of monoterpene. In Fig. 2a , we show the loss rate of the p-HOM-RO 2 at different NO levels. NO has a non-linear influence on the loss rate of the p-HOM-RO 2 and thus the possibility that p-HOM-RO 2 becomes HOM-RO 2 . When NO is absent, p-HOM-RO 2 loss is primarily due to the cross-reaction with non-HOM-RO 2 (defined as RO 2 that cannot autoxidize). Low but non-zero NO (e.g., 10 pptv) drastically reduces the total loss rate of p-HOM-RO 2 by efficiently reducing the concentration of non-HOM-RO 2 . Although NO also consumes p-HOM-RO 2 , at low NO this effect is more than compensated by the decrease in non-HOM-RO 2 , which dominates the loss of p-HOM-RO 2 at this NO level. As the NO concentration further increases, it progressively becomes the dominant sink of the p-HOM-RO 2 (Fig. 2a ) and starts to inhibit HOM production. This intervention in the RO 2 cross-reactions can also partially explain the suppression effect of NO 2 on HOM formation, in addition to the termination of chain propagation of acyl RO 2 [31] . Elevated NO 2 produces considerable non-HOM-RO 2 via NO 3 oxidation, which reduces the probability of p-HOM-RO 2 producing HOM. Fig. 2: The mechanism through which NO can enhance the formation of highly oxygenated organic molecules (HOM) from monoterpene oxidation at 278 K. ( a ) Loss rates of p-HOM-RO 2 (RO 2 that can undergo autoxidation with n O < 7) as a function of NO concentration in the varying NO/NO 2 experiment. Reactions of RO 2 + HO 2 , RO 2 + NO, and RO 2 + RO 2 are marked by pink, blue, and red, respectively. ( b ) The fraction of p-HOM-RO 2 that can undergo autoxidation to HOM-RO 2 with (the sum the blue and green fillings) and without (green fillings) NO-induced RO autoxidation in the varying NO/NO 2 experiment. ( c ) Comparison between HOM yields with (solid blue line) and without NO (dashed green line) RO autoxidation. In the simulation of Fig. 2c , the concentrations of monoterpene, O 3 , and NO 2 are constrained at 1200 pptv, 40 ppbv and 1 ppbv. Full size image Aside from modulating the HOM-RO 2 loss rate, NO also affects the formation of HOM-RO 2 directly by converting RO 2 to RO. As studied under high-NO conditions [35] , a fraction of RO can isomerize and form new RO 2 via intra-molecular hydrogen abstraction followed by instantaneous O 2 addition. In the context of HOM formation, we refer to RO isomerization as the “RO autoxidation channel” (Supplementary Fig. 5 ), as it is similar to the definition of RO 2 autoxidation. It should be noted that the RO autoxidation channel has been shown to play a non-negligible role in HOM formation following α-pinene ozonolysis under NO x -free conditions, as RO 2 cross-reactions also lead to RO formation [36] . But the presence of NO leads to additional RO formation, making this channel more important. In the case of alkane photo-oxidation, which can have very low yields of highly oxygenated products, the addition of NO was recently shown to greatly enhance the concentration of the most oxygenated products [37] . This was inferred to be due to several steps of RO isomerization taking place, causing the efficient formation of highly oxygenated species even at 10 ppbv NO. We cannot directly measure the short-lived RO radicals, so we use distinct HOM products as markers to examine the importance of this channel. In the ozonolysis of monoterpenes, HOM-RO 2 produced via direct autoxidation contain an odd number of hydrogen atoms ( n H ) and an even number of oxygen atoms ( n O ), e.g., C 10 H 15 O 8,10 . The corresponding closed-shell HOM from either unimolecular termination or bimolecular reactions with RO 2 and HO 2 must be C 10 H 14,16 O 7,9 and C 10 H 16 O 8,10 (Supplementary Fig. 5 ), which are the major HOM products in many experiments without NO x [6] , [36] , [38] . In contrast, RO isomerization will produce an RO 2 with an odd n O , and the consequent closed-shell species are e.g. C 10 H 14 O 8,10 (Supplementary Fig. 5 ). In Supplementary Fig. 6 , we show the variation of C 10 H 14 O 8,10 at different NO levels. As NO rises, they increase by ca . 30 and 100 %, respectively, illustrating the enhancement of the RO autoxidation channel (Fig. 2b ). In Fig. 2c , we show the importance of RO autoxidation by comparing the results with and without this reaction channel. The ADCHAM model can only reproduce the experimental data when the RO reaction channel is implemented. Without the RO reaction channel, the predicted HOM yield is significantly lower than the experimental observation, and the difference diverges at higher NO concentrations. This channel forms ca . 25% of HOM even at only 10 pptv NO, and it is responsible for almost all the HOM formation at above 100 pptv NO. Because of this, the HOM yield remains at a considerable level at high NO concentration, although still lower than the yield under NO-free conditions. It is worth noting that RO autoxidation also explains the large fraction of CHO-HOM formed with the direct involvement of NO (Supplementary Fig. 2 ). We summarize the dependences of HOM yields on NO and NO 2 in Fig. 3 . In general, NO 2 suppresses HOM production monotonically, and NO has a non-linear effect (Fig. 3a ). It was previously thought that HOM suppression by NO 2 was mostly due to the direct reaction of RO 2 + NO 2 outcompeting RO 2 autoxidation [32] . However, we find that NO 2 can suppress HOM production indirectly by increasing the loss rate of HOM-RO 2 - it promotes NO 3 -initiated monoterpene oxidation, which forms a considerable amount of non-HOM-RO 2 , enhancing the second-order RO 2 cross-reactions. When NO is also present, it counteracts the suppression effects of NO 2 : on the one hand, it can significantly consume NO 3 ; on the other hand, it reduces the total loss rate of HOM-RO 2 (Fig. 2a ). Our results suggest that the highest HOM yield at different NO 2 levels is similar when NO is present, although the optimal NO concentration varies slightly. This makes the enhancement of HOM yield by NO more significant at high NO 2 (up to 140% with NO 2 at 10 ppbv, Fig. 3a ). The enhancement of HOM yield at low NO is pronounced for CHO HOM at low NO 2 concentrations (e.g., <5 ppbv) (Fig. 3b ) and for CHON HOM at high NO 2 concentrations (e.g., >5 ppbv) (Fig. 3c ). Fig. 3: Model simulated non-linear dependence of the yields of highly oxygenated organic molecules (HOM) on NO 2 and NO at 278 K. ( a ) total HOM, ( b ) CHO-HOM, and ( c ) CHON-HOM with 1200 pptv monoterpene. O 3 concentrations are constrained at 40 ppbv at each experiment. The contour lines indicate the corresponding HOM yields. Full size image It is worth noting that the quantitative relationships outlined here may be sensitive to conditions in human-influenced environments, where a greater abundance of non-HOM-RO 2 originating from small molecule VOCs may lead to a stronger loss of HOM-RO 2 . In this case the maximum HOM yield is expected to occur at a higher concentration of NO. Atmospheric observational evidence and implications We demonstrate that HOM formation is governed by a complex competition between multiple reactions including RO 2 autoxidation, RO isomerization, and various uni-molecular and bi-molecular termination reactions. Therefore, HOM yields vary depending on NO, NO 2 , and monoterpene concentrations and are expected to vary significantly in different environments rather than remain constant. As shown in Fig. 4 , we reproduce the HOM yields in a boreal forest in southern Finland by implementing these insights. The details of the simulation inputs and assumptions are provided in Methods. The calculated HOM yield as a function of measured NO x and monoterpene concentrations varies by almost a factor of three, from 2.5% to 6.5%. This large variation can cause a notable change in both SOA formation and particle growth. Fig. 4: Contour plot of the yields of highly oxygenated organic molecules (HOM) from monoterpene oxidation vs monoterpene and NO x concentration. The observation data of monoterpene and NO x from the SMEAR II boreal forest station [58] are used to predict the HOM yield (black points). A series of simulations were conducted with monoterpene concentration varying from 100 to 1800 pptv, and NO x concentration from 0.01 to 100 ppbv. With the assumption NO is solely formed from NO 2 photolysis, NO/NO 2 varied to follow the observed diurnal cycle at SMEAR II station from almost zero at night to 14.3% at 10 am. We take the daytime average HOM yield as the HOM yield at fixed NO x and monoterpene concentration. Full size image Although this study investigates HOM formation at low and moderate NO levels, the highlighted importance of the RO autoxidation channel also advances our understanding of HOM formation at high NO concentrations, common for monoterpene oxidation in the polluted urban boundary layer. It has been argued that HOM formation can be completely suppressed when the RO 2 + NO reaction overwhelms RO 2 autoxidation [15] . However, our measurements in polluted East China show that the HOM yield of monoterpene oxidation remains at approximately 1–2% on average (Supplementary Fig. 7 ), instead of approaching zero as anticipated. This discrepancy can be explained by RO autoxidation, as we demonstrated in Fig. 2c . Besides monoterpene oxidation, the RO autoxidation channel should be important in the oxidation of other VOCs, such as alkanes [8] , [37] . This is consistent with the significant anthropogenic HOM production observed in polluted megacities with high NO concentrations [8] . We conclude that high NO cannot completely inhibit HOM formation even in severely polluted urban environments. In summary, combining experimental data, ambient observations, and molecule-level model simulations, we demonstrate that NO has a non-linear effect on HOM formation. Though NO x maxima are known for phenomena such as O 3 production and HO x concentrations, the maxima occur at different points. For HOM production, the maximum is at very low NO, meaning that environments can be “low NO x ” for O 3 yet “high NO x ” for HOM. 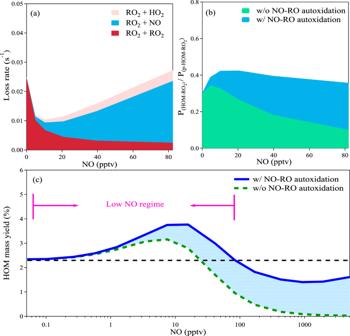Fig. 2: The mechanism through which NO can enhance the formation of highly oxygenated organic molecules (HOM) from monoterpene oxidation at 278 K. (a) Loss rates of p-HOM-RO2(RO2that can undergo autoxidation withnO< 7) as a function of NO concentration in the varying NO/NO2experiment. Reactions of RO2+ HO2, RO2+ NO, and RO2+ RO2are marked by pink, blue, and red, respectively. (b) The fraction of p-HOM-RO2that can undergo autoxidation to HOM-RO2with (the sum the blue and green fillings) and without (green fillings) NO-induced RO autoxidation in the varying NO/NO2experiment. (c) Comparison between HOM yields with (solid blue line) and without NO (dashed green line) RO autoxidation. In the simulation of Fig.2c, the concentrations of monoterpene, O3, and NO2are constrained at 1200 pptv, 40 ppbv and 1 ppbv. We propose a new division of NO regimes including “Zero NO x ”, “Low NO”, and “High NO” (Supplementary Table 2 ) in HOM-related studies. In this new division, previous studies almost completely overlooked the low-NO regime, in which HOM formation is enhanced due to a reduced sink of HOM-RO 2 as well as enhanced RO autoxidation. Conceptually, this non-linear effect is similar to the radical termination via production of organonitrates (at intermediate NO x ) [39] and even the catalytic ozone depletion in the stratosphere (with NO x suppressing HO x and ClO x catalysis at low concentrations but ultimately enhancing catalytic ozone loss at sufficiently high NO x ) [40] . All these reveal the notably different outcomes between low-concentration and high-concentration reactions in atmospheric photochemistry. In fact, from a global perspective, high-NO environments are the exceptions, existing only near the ground surface of regions with strong human activity, whereas low-NO environments likely prevail in the vast majority of Earth’s boundary layer. As shown in Supplementary Fig. 8 , the low-NO regime (NO < 30 pptv) prevailed at our boreal-forest reference site, accounting for more than half of the observation period from 2002 to 2018. In a megacity of east China, although only 6% of the observation data was lower than 30 pptv, the frequency of low-NO conditions has increased significantly in recent years due to NO x emission controls. Therefore, this refined understanding of HOM formation in the low-NO regime is crucial for an accurate evaluation of HOM and aerosol budgets, as well as climate change. The CLOUD chamber The CLOUD chamber is a well-controlled stainless-steel cylinder with a volume of ca. 26.1 m 3 , located at CERN, Geneva, Switzerland [28] , [41] . Plenty of efforts were made to keep the chamber ultra-clean, including using an electro-polished inner surface, rinsing with 373 K ultrapure water and flushing the chamber with humidified synthetic air containing several ppmv of ozone thereafter before each campaign. Synthetic air used throughout the campaign was produced by mixing ultra-clean cryogenic liquid nitrogen and oxygen. These efforts achieved an as low as possible contamination level that the background VOCs concentration is below ppbv level and the condensable vapors are mostly below the detection limits, and allowed investigating the chemical processes with atmospherically relevant concentration of reaction precursors [42] , e.g. pptv level monoterpene and NO x . It is worth noting that with the ultra-clean electro-polished stainless-steel surface, the influence of HO 2 produced from the chamber wall which was a long-standing trouble for Teflon chambers is believed to be ignorable during the campaign. Several light system covering different regions of the UV and visible spectrum was equipped in the chamber to simulate the atmospheric photochemistry, including a Krypton-Fluoride excimer UV-laser (3 W, λ = 248 nm), two UV LEDs (2 × 16.5 W, λ = 370–390 nm) and four Hamamatsu Xenon arc lamps (4 × 200 W, λ = 250–580 nm) [9] , [43] . For varying NO/NO 2 experiment run during CLOUD11, an additional UV-sabre (400 W UVS3, centered on 385 nm) system was installed to further photolyze NO 2 into NO. The NO/NO 2 ratio can be adjusted by changing the UV-sabre light intensity. The NO 2 photolysis frequency, jNO 2 , was measured by NO 2 actinometry and varying the UV-sabre intensity. Experimental design Our objective of this study is to investigate the role of NO x in the oxidation of monoterpene and HOM formation in the atmospherically relevant concentrations (low NO x environment). The chamber conditions were kept stable at the temperature of 278 K and relative humidity of 38%. Ozone was injecting at a constant rate to keep the concentration around 40 ppbv. The monoterpene used in this study is a mix of α-pinene and Δ−3-carene with a volume mixing ratio of 2:1, which represents the condition at our reference site of SMEAR II station in southern Finland [29] , [30] . The steady-state concentration of monoterpene mixture was set to 300 pptv, 600 pptv and 1200 pptv. In this study, with the target to understand the role of NO x in detail, we conducted three different experiment runs, including pure NO 2 run, constant NO/NO 2 ratio runs and, varying NO/NO 2 run. Pure NO 2 run and constant NO/NO 2 ratio runs were conducted during November of 2015 (CLOUD10 campaign). The varying NO/NO 2 experiment was performed in November of 2016 (CLOUD11 campaign). NO 2 was injected into the chamber under dark condition during pure NO 2 run to maintain a NO free environment. NO was injected into the chamber for constant NO/NO 2 runs, and mostly oxidized to NO 2 by reacting with O 3 . For each experiment run, monoterpene was injected into the chamber to get its steady-state concentration before injecting NO x . The steady-state concentrations of NO x were set to 0, 0.7, 1.9 and 4.6 ppbv for the pure NO 2 run and constant NO/NO 2 ratio runs, representing very clean to slightly polluted environments, and at approximately 1 ppbv for the varying NO/NO 2 experiment to represent the mean value at the SMEAR II station. Throughout all the NO/NO 2 experimental runs, the UV LEDs light system was kept on to photolyze some NO 2 to NO. The ratio of NO/NO 2 was kept at ~0.7% in constant NO/NO 2 experimental runs. Noting that due to the titration of NO in the NO injection run (constant NO/NO 2 experiment), the steady state concentration of O 3 decreased slightly from 40 ppbv at 0 ppbv NO x to around 36 ppbv at 4.6 ppbv NO x . During the varying NO/NO 2 experimental run, NO concentration was adjusted from 0 pptv to 82 pptv by changing the intensity of UV-sabre. Measurements Measurement of gas-phase HOM and OH radicals. Concentrations of highly oxygenated molecules (HOM) were measured with a nitrate-ion based chemical ionization atmospheric pressure interface time-of-flight mass spectrometer (CI-APi-TOF) [44] . The nitrate ions are produced by exposing nitric acid (HNO 3 )-containing sheath flow to soft x-ray radiation. The sulfuric acid and targeted HOM are charged in the drift tube before entering to the APi and analyzing in the TOF chamber. To quantify HOM, the system was calibrated and corrected using the methods similar to our previous work [9] , [10] . Since the loss rate of sulfuric acid is well characterized, the concentration and calibration coefficient can be obtained. This calibration coefficient was also used to quantify HOM with the consideration of weight-dependent ion transmission [45] and sampling loss in the inlet. We processed the raw data using the MATLAB tofTools package (version 603) [44] . High-resolution analysis was used to identify the peaks with different elemental formulae. OH concentrations in the chamber were determined by the following equation. [OH]=k_loss[SA]/k_SO2+OH[OH]× [SO_2]
 (1) Where k loss refers to the loss of sulfuric acid to the aerosol particles (condensation sink) and to the wall (wall loss); k SO2+OH refers to the reaction rate constant between OH and SO 2 at 278 K. OH concentrations were also simulated by the ADCHAM model. The simulated concentration was identical to the estimated concentration via Eq. ( 1 ). NO 3 concentrations were calculated by the change in monoterpene concentration after adjusting NO x concentration at each experimental steps. Measurement of monoterpenes and trace gases. A newly developed proton transfer reaction time-of-flight mass spectrometer, named PTR3, was deployed to measure the concentrations of monoterpenes and other VOCs [46] . Since α-pinene and Δ−3-carene fragment differently in the instrument, they can be calibrated individually. Sulfur dioxides (SO 2 ) and ozone (O 3 ) were measured using Thermo Scientific gas monitors (model 42i for SO 2 and model 49i for O 3 ). In view of the low concentration of nitrogen oxide (NO), an advanced NO monitor (ECO PHYSICS, model: CLD 780 TR) was used to measure NO accurately. The detection limit of this NO monitor is 3 pptv for 1-min integration time. Nitrogen dioxide (NO 2 ) was measured using a cavity-attenuated phase-shift nitrogen dioxide monitor (CAPS NO 2 , Aerodyne Research Inc.) close to the injection of the chamber and by Cavity-Enhanced Differential Optical absorption spectroscopy (CE-DOAS) at the top of the chamber. NO and NO 2 were injected at the bottom of the chamber close to a mixing fan and quickly dispersed into the chamber. NO 2 measurements at the top and bottom of the chamber suggest the NO 2 concentrations to be well mixed, with concentrations at the top and bottom typically not differing by more than 25%. All the gases were sampled from the middle of the chamber. For the NO 2 injection runs, including the pure NO 2 experiment run and the varying NO/NO 2 experiment run, all the trace gases were homogeneous distributed in the chamber. For the constant NO/NO 2 experiment runs, the NO mixing ratio close to its injection port was about 5 times higher than that in the middle of the chamber. However, due to the fast reaction of NO and O 3 , the space with highly concentrated NO should be much smaller than the overall chamber volume. Ambient measurement campaigns of HOM. Ambient HOM measurement data from two field campaigns were used to verify the role NO x in HOM formation in the real atmosphere. One campaign was conducted at a boreal forest site (SMEAR II station) in southern Finland between 15 and 24 May 2013 to represent the low-NO x environment [11] , and the other was at an urban site in east China (SORPES station) during 2 August and 6 September 2019 to represent the high-NO x environment [22] . Detailed description of the campaigns can be found in Roldin et al., 2019 [11] and Liu et al., 2021 [22] . In short, a CI-APi-HTOF at SMEAR II and a CI-APi-LTOF at SORPES were used to measure HOM and sulfuric acid. VOCs precursors were measured by a proton transfer reaction mass spectrometer (PTR-MS, Ionicon). NO x and other trance gases (e.g., O 3 ) were measured by TEI gas analyzers. Positive matrix factorization (PMF) PMF is a widely used receptor model for source apportionment analysis [47] . In this study, we first preformed the high-resolution peak fitting for the varying NO/NO 2 experiment run, during which an LToF based nitrate CIMS was deployed with the resolution up to ~10,000 Th/Th that allowed us to identify the peaks more accurate. Then, we prepared the data matrix and error matrix according to the methods described by Yan et al. [17] for the PMF model input. An IGOR based analyzing interface SoFi (solution finder, version6.3) and ME-2 was used to perform the high-resolution PMF analysis [48] . A detailed description of PMF used for a nitrate-CIMS based dataset can be found in our previous study [17] . 5 factors resolved from the PMF analysis provide the optimal solutions. We shortly introduce the 5 factors as follows. Δ−3-carene ozonolysis factor (D3C factor): 400 pptv Δ−3-carene was injected into the chamber as the first run-step, during which only carene and ozone reacted in the chamber. Therefore, PMF resolved the Δ−3-carene ozonolysis factor as the first factor, the spectrum of which is a bit different from the well-known α-pinene ozonolysis factor (Supplementary Fig. 3 ) [6] . The pre-dominant molecule is C 10 H 14 O 9 , followed by two RO 2 radicals of C 10 H 15 O 8 and C 10 H 15 O 10 . Dimer formation at this stage is not significant, due to the lower concentration of precursors which that limit the RO 2 cross-reactions. α-pinene and Δ−3-carene ozonolysis factor (AP + D3C factor): 800 pptv α-pinene was added after the Δ−3-carene step reaching the steady state to obtain the targeted mixture of monoterpenes. PMF identified this system as a pure ozonolysis factor, the spectrum of which is very similar to Nighttime Factor 1 resolved from field observation at SMEAR II station (Fig. S4 ) [17] . Compared to the D3C factor, the intensity of C 10 H 14 O 7 increased dramatically and was to be one of the main fingerprint molecules of the AP + D3C factor. In contrast, RO 2 radicals (e.g., C 10 H 15 O 8 and C 10 H 15 O 10 ) decreased significantly, probably due to the enhanced RO 2 cross-reactions which consumed RO 2 radicals but promoted the dimer formations, e.g., C 19 H 28 O 11 and C 20 H 32 O 11 . In addition, the intensity of OH-initiated HOM molecules, e.g., C 10 H 16 O 7 and C 10 H 16 O 9 , enhanced significantly. It could be that OH production from monoterpene ozonolysis was elevated, or the HOM yield from OH oxidation of α-pinene was higher than OH oxidation of Δ−3-carene. NO 3 oxidation factor (NO 3 factor): Around 1 ppb NO 2 was injected into the chamber after the above two steps. NO 2 reacted with O 3 to form NO 3 radical, which oxidized monoterpenes to be an additional HOM source. Therefore, PMF resolved an NO 3 factor aside from the pure ozonolysis factor at this stage. The spectrum of the NO 3 factor was similar to that of the Nighttime Factor 2 resolved from field observation at SMEAR II station (Fig. S4 ) [17] . CHON monomers of C 10 H 15 O 8,10 N and dimers of C 20 H 31 O 11,13 N were the major fingerprint molecules. A significant formation of C 10 H 16 O 10 N 2 was observed at this stage (in the NO 3 factor), during which only NO 3 and NO 2 presented as the N-containing precursor gases. This is different from previous understanding that CHON 2 can be only formed from a CHON radical produced from NO 3 oxidation and terminated by NO. One possible explanation is that C 10 H 16 O 10 N 2 in this factor is acyl nitrate formed via the reaction of an acylperoxy radical with NO 2 . NO involved NO 3 oxidation factor (NO 3 + NO factor): After producing NO by photolyzing NO 2 in the chamber, a new factor was resolved and defined as NO 3 + NO factor (Supplementary Fig. 3 ). This factor is a transition factor from the NO 3 factor to a NO heavily participating factor (NO factor). A bunch of CHON molecules, e.g., C 10 H 15 O 7 N and C 10 H 15 O 9 N, were formed from the reaction between RO 2 radical and NO. Additional CHON 2 molecules other than C 10 H 16 O 10 N 2 , e.g., C 10 H 16 O 9 N 2 , were formed from the NO 3 -initiated CHON radical reacting with NO. Dimer formation became very week. Fragmented molecules (e.g., C 5 H 6 O 7 ), as well as C 15 HOM molecules (e.g., C 15 H 17 O 9,10 ), started to appear in this factor because of the NO, which can react with RO 2 to form RO to enhance the possibility of fragmentation. NO heavily participating factor (NO factor): When further stepping up the NO concentration, PMF resolved another factor, in which NO participated the HOM formation heavily (Supplementary Fig. 3 ). In this factor, a considerable amount of fragmented molecules (e.g., C 5 H 6 O 5 , C 5 H 6 O 7 , C 7 H 11 O 8 , and C 8 H 13 O 9 N) were observed. HOM dimers almost disappeared, suggesting the reaction with NO was becoming the dominating fate of RO 2 instead of its cross-reaction. In summary, optimal PMF solutions provide 4 types of factors for all the four experimental runs, including two ozonolysis factors (D3C factor and MT factor), an NO 3 oxidation factor (NO 3 factor), an NO involved NO 3 oxidation factor (NO 3 + NO factor) and a NO heavily-participating factor (NO factor). Factors appear successively from the D3C factor to the NO factor accompanying with stepping up of NO 2 or NO. The spectrum of HOM changes as follows: it is dominated by typical CHO HOM in the ozonolysis factors, but switches to CHON monomers (e.g., C 10 H 15 O 8,10 N) and dimers (e.g., C 20 H 31 O 11,13 N) in NO 3 factor. In the NO 3 + NO factor, CHON (e.g., C 10 H 15 O 7-10 N) dominates and CHON 2 (e.g., C 10 H 16 O 9,10 N 2 ) appears extensively. Finally, a significant amount of fragmented molecules (e.g., C 5 H 6 O 5 , C 5 H 6 O 7 , C 7 H 11 O 8 ) appears in the NO factor. HOM dimers decreases gradually and almost disappear in the NO factor. This is in accordance with our previous understanding that CHON radicals and CHON dimers can be only formed from the NO 3 involved reaction chain; most CHON 2 are only formed from a CHON radical produced from NO 3 oxidation and terminated by NO, except for some acyl nitrate formed via the reaction of an acylperoxy radical with NO 2 (e.g., C 10 H 16 O 10 N 2 ). ADCHEM model We use the Aerosol Dynamics gas- and particle-phase chemistry model for laboratory CHAMber studies (ADCHAM) [49] and the trajectory model for Aerosol Dynamics gas- and particle-phase CHEMistry and radiative transfer (ADCHEM) [50] . They share a detailed gas-phase kinetic code that combines peroxy radical autoxidation mechanism (PRAM) and Master Chemical Mechanism version 3.3.1 (MCMv3.3.1) using the Kinetic PreProcessor (KPP) [51] . As described in Roldin et al., 2019 [11] , PRAM explicitly simulates the formation of peroxy radicals (RO 2 ) and their oxidation products. 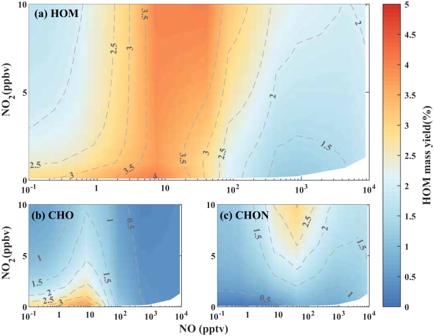Fig. 3: Model simulated non-linear dependence of the yields of highly oxygenated organic molecules (HOM) on NO2and NO at 278 K. (a) total HOM, (b) CHO-HOM, and (c) CHON-HOM with 1200 pptv monoterpene. O3concentrations are constrained at 40 ppbv at each experiment. The contour lines indicate the corresponding HOM yields. 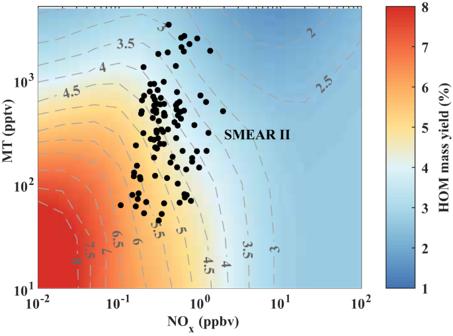Fig. 4: Contour plot of the yields of highly oxygenated organic molecules (HOM) from monoterpene oxidation vs monoterpene and NOxconcentration. The observation data of monoterpene and NOxfrom the SMEAR II boreal forest station58are used to predict the HOM yield (black points). A series of simulations were conducted with monoterpene concentration varying from 100 to 1800 pptv, and NOxconcentration from 0.01 to 100 ppbv. With the assumption NO is solely formed from NO2photolysis, NO/NO2varied to follow the observed diurnal cycle at SMEAR II station from almost zero at night to 14.3% at 10 am. We take the daytime average HOM yield as the HOM yield at fixed NOxand monoterpene concentration. We provide the yield, branch ratio, and autoxidation rate constants of main chemical reactions in Supplementary Table 3 . Given that the mechanism of fragmentation chemistry is not well understood, ADCHAM tends to underestimate the fragments, the production of which is accompanied by an increase in the NO/MT ratio. Therefore, the model slightly underestimates the HOM yield in the highest NO x step of the constant NO/NO 2 experiment with 300 pptv monoterpene (Fig. 1c ). In this work, we added the following mechanisms into the model to improve the simulation. (1) NO 3 chemistry in HOM formation, which included RO 2 formed when monoterpenes are oxidized by NO 3 and RO formed via RO 2 -NO 3 reactions. (2) Terminal reaction by bimolecular reactions between NO 2 and certain RO 2 (e.g., C 10 H 15 O 5 ) (3) Various isomers of RO 2 were considered, which greatly reduced the uncertainty of simulating responses that are highly dependent on RO 2 structures. (4) Refine the representation of RO isomerization Since HOM have very low saturation vapor pressures, we assume that they are lost losses irreversibly onto the chamber wall, and calculate the wall loss from the following equation [52] : 
    k_wall= C_wall√(D)
 (2) where C wall is an empirical parameter, which is 0.0075 cm −1 s −0.5 derived from dedicated sulfuric acid decay experiments at 5 °C. The diffusion coefficients D i for each HOM i are approximated with the equation \({{{{{{\rm{D}}}}}}}_{{{{{{\rm{i}}}}}}}({{{{{{\rm{cm}}}}}}}^{2}{{{{{{\rm{s}}}}}}}^{-1})=0.31\bullet {{{{{{\rm{M}}}}}}}_{{{{{{\rm{i}}}}}}}^{-1/3}\) , where M i is the mass of molecule with the unit of g mol −1 . HOM yield calculation HOM yield calculation in CLOUD chamber and SMEARII station: we defined the yield of HOM as the fraction of reacted monoterpenes that produced HOM. Due to the complex formation of HOM through multiple oxidations, the production rate of HOM was replaced by the HOM loss rate under steady state: 
    MT-HOM  yield=k_loss[HOM]/k_MT+oxidants[oxidiants]× [MT]
 (3) where oxidants consist of O 3 , OH, and NO 3 in this study and k loss is the total loss rate of HOM to the chamber walls in CLOUD experiments, to the ground or other surfaces (Dry deposition) and aerosol particles (condensation) in field observations. We propagate the error for each chamber experiment with four different NO x levels. Within each selected time windows, absolute errors of [HOM], [SO 2 ], [sulfuric acid], CS, [O 3 ], [α-pinene], [Δ−3-carene] are derived from the measurements as the 3-sigma standard deviation. Since NO 3 concentrations are calculated based on the consumed monoterpene concentration, they share the same relative error with [α-pinene] and [Δ−3-carene]. For the loss of HOM, we assume zero error for k wall and k dilu . The propagated error of the HOM yield varies slightly within 6–8% among different experiments (Fig. 1 ). When calculating condensation for HOM measured at SMEAR II, pure liquid saturation vapor pressures( p 0 ) were calculated based on saturation concentrations (C sat ), which can be parameterized by the numbers of carbon(n C ), oxygen(n O ), and nitrogen(n N ) atoms [53] : 
    log_10(C_sat)=(n_0-n_C)b_C-(n_O-3n_N)b_O-2(n_O-3n_N)n_C/(n_C+n_O-3n_N)b_CO-n_Nb_N
 (4) where n 0 = 25, b C = 0.475, b O = 0.2, b CO = 0.9, and b N = 2.5, respectively. As volatilities of organic molecules detected span over a wide range, we grouped the hundreds of organic molecules detected in the chamber into different bins within a volatility basis set (VBS) [54] . Then we can calculate the HOM mass yield via formula (3), in which monoterpene concentrations were measured, HOM was also measured and grouped into a series of bins, k loss , OH and NO 3 radical were simulated by the model. To minimize the potential uncertainty, we selected HOM species with C*(300 K) below 3×10 −4 μg m −3 as those would condense onto aerosol particles irreversibly. HOM yield calculation at SORPES station: In polluted east China, where VOCs species distribution and photochemistry are far more complex than in the boreal environment, it is challenging to simulate HOM concentrations. Especially during nighttime, when the NO concentration is very high and consume most known oxidants, e.g., NO 3 radical and O 3 . Therefore, we only calculated the daytime HOM yield through the following Eq. ( 5 ): 
    MT-HOM  yield=[ELVOCs]_MT·CS/k_MT+OH[MT]·[OH]+k_MT+O_3[MT]·[O_3]
 (5) Here, \({[{{{{{\rm{ELVOCs}}}}}}]}_{{{{{{\rm{MT}}}}}}}\) is the concentration of monoterpene-derived ELVOCs, \(\left[{{{{{\rm{MT}}}}}}\right]\) is the concentration of monoterpenes. Monoterpene derived HOM are selected as HOM molecules with a carbon number of 10 and a double bond equivalent (DBE) number between 2 and 4 [8] . Since the atmospheric oxidation capacity in polluted east China is usually strong, HOM are possibly produced through multi-generational oxidation. We estimated the contribution of multi-generation by the following method, and excluded it from the yield calculation. First, dinitrates (HOM molecules with two nitrate groups) are regarded as the multi-generational products, since one oxidation step can only add one nitrate group to the product molecule; Second, HOM molecules with a DBE of 2 are produced either from OH-initiated oxidation of monoterpenes or from the multi-generational oxidation process of monoterpenes. The calculated contribution of multi-generational oxidation to monoterpene HOM ranges from 15.8% to 33.5%. Here, we only selected non-nitrates and mononitrates with a DBE of 3−4 to calculate the yield to exclude the effects of multi-generational oxidation (Supplementary Fig. 7 ). Molecules with C*(300 K) of below 3×10 −4 μg m −3 were further selected as ELVOCs those can condense onto aerosol particles irreversibly. Since the oxidation products with higher volatility are not included due to their long lifetimes cause the steady-state assumption not to hold, the HOM yield calculated here, which is considerably under-estimated, can be considered as the low limit. The OH concentration was calculated by applying the Eq. ( 1 ), based on the assumption that gaseous sulfuric acid is mostly produced from the oxidation of SO 2 by OH and primarily lost by condensing onto particles. \({{{{{{\rm{k}}}}}}}_{{{{{{\rm{OH}}}}}}+{{{{{{\rm{SO}}}}}}}_{2}}\) is a termolecular reaction constant for the rate-limiting step of the formation pathway of H 2 SO 4 at the temperature of the sampling time in the atmosphere [55] , and k loss is the loss rate of H 2 SO 4 by condensation to aerosol surface (CS, condensation sink). Although reactions of SO 2 with products from the ozonolysis of alkenes generate a moderate amount of nighttime sulfuric acid, with little effect on daytime sulfuric acid [56] . This is also one reason that we calculated the yield of MT-HOM only during the daytime in this study. The error of OH does not change the relative distribution of RO 2 from different precursors. In the atmosphere without direct anthropogenic emissions, NO concentrations, mainly from the photolysis of NO 2 , show a clear diurnal cycle from almost zero during the night to its maximum before noontime. For example, NO concentration and NO to NO 2 ratio revealed its peak value at around 10:00–11:00 am at our reference station of SMEAR II [17] . Correspondingly, the HOM yield will vary non-linearly and diurnally. Therefore, the HOM yield is determined by the ratio of NO/NO 2 at a specific time of the day. We thus take the daytime average HOM yield as the HOM yield at fixed NO x and monoterpene concentration. We conducted a series of simulations with monoterpene concentration varying from 100 to 1800 pptv, and NO x concentration from 0.01 to 100 ppb. With the assumption NO is solely formed from NO 2 photolysis, the NO/NO 2 ratio varied to follow the observed diurnal cycle at SMEAR II station from almost zero at night to 14.3% at 10 am. The average daily dependence of HOM on monoterpene and NO x concentrations can be estimated on the basis of integration with this function. We then take the daily average HOM yield as the HOM yield at fixed NO x and monoterpene concentration, and illustrated in Fig. 4 .